Transplanted terminally differentiated induced pluripotent stem cells are accepted by immune mechanisms similar to self-tolerance The exact nature of the immune response elicited by autologous-induced pluripotent stem cell (iPSC) progeny is still not well understood. Here we show in murine models that autologous iPSC-derived endothelial cells (iECs) elicit an immune response that resembles the one against a comparable somatic cell, the aortic endothelial cell (AEC). These cells exhibit long-term survival in vivo and prompt a tolerogenic immune response characterized by elevated IL-10 expression. In contrast, undifferentiated iPSCs elicit a very different immune response with high lymphocytic infiltration and elevated IFN-γ, granzyme-B and perforin intragraft. Furthermore, the clonal structure of infiltrating T cells from iEC grafts is statistically indistinguishable from that of AECs, but is different from that of undifferentiated iPSC grafts. Taken together, our results indicate that the differentiation of iPSCs results in a loss of immunogenicity and leads to the induction of tolerance, despite expected antigen expression differences between iPSC-derived versus original somatic cells. Pluripotent stem cells (PSCs) can be artificially generated in vitro by introducing a combination of defined factors into somatic cells [1] , [2] . These cells, termed as induced PSCs (iPSCs), can differentiate into any somatic cells essentially and thus hold exceptional potential as sources of therapeutic cells for personalized medical applications such as organ repair. From an immunological standpoint, this technology brings tremendous benefits because patients could be treated with autologous cells, thereby avoiding life-long immunosuppressive therapy currently required for preventing rejection of allografts, which is costly and associated with significant side effects. However, the unexpected immunogenicity of syngeneic iPSCs demonstrated by a previous study [3] raised serious concerns about the value of these iPSCs as a source of autologous cellular therapeutics. Slight differences in antigen repertoire introduced by neoantigens arising from genomic alterations acquired during the reprogramming process, or during the differentiation of iPSCs into the desired tissue, can profoundly alter the immunogenicity profiles [4] , [5] , [6] , [7] . Hence, a thorough assessment of the immunological phenotype elicited by tissues derived from iPSCs is essential before the potential translation of this technology into clinics. In this study, we sought to delineate the impact of terminal differentiation of iPSCs on immunogenicity of their progeny using a mouse model of autologous transplantation, and to determine how closely the immunological phenotype elicited by these cells relates to that of corresponding self-somatic cells. We show that autologous endothelial tissues derived from iPSCs can elicit an immune response that resembles the one against self, as represented by the aortic endothelial cells (AECs). These cells exhibited long-term survival in vivo and elicited an immune contexture consistent with self-tolerance. By contrast, autologous undifferentiated iPSCs were rejected with hallmark features of lymphocytic infiltration accompanied by abundant expression of interferon-γ (IFN-γ) and cytotoxic factors (granzyme-B and perforin). To further examine the immunological relatedness among iECs, AECs and undifferentiated iPSCs, we used high-throughput T-cell receptor (TCR) sequencing analysis and found that the clonal structure of infiltrating T cells found in iEC grafts was statistically indistinguishable from that of AEC grafts, but was clearly different from that of undifferentiated iPSC grafts. Taken together, our results demonstrate that differentiation of iPSCs could result in a loss of immunogenicity and in immunological responses that are similar to the one elicited by a corresponding self-somatic cell. Murine iPSCs are rejected in syngeneic recipients In order to determine the survival kinetics of iPSCs in vivo , fibroblasts from transgenic FVB mice ubiquitously expressing green fluorescence protein and luciferase (GFP.Luc + ) were used to generate iPSC lines using two approaches. Reprogramming of fibroblasts was performed using a lentiviral (LV)-based or a minicircle plasmid-based approach (genome-integration free) for delivery of the four reprogramming factors (Klf4, Oct4, Sox2 and c-Myc) as described elsewhere [1] , [8] . The resulting iPSCs were characterized for pluripotency ( Supplementary Fig. 1 ) and their immunogenicity was assessed in syngeneic versus immunodeficient recipients. Transgenic expression of the luciferase reporter gene allowed tracking of iPSCs in vivo by bioluminescence imaging (BLI) over the course of the experiment. Mouse iPSCs (1 × 10 6 ) were implanted intramuscularly in the legs of syngeneic FVB mice. BLI tracking of cell survival revealed a complete loss of bioluminescence in both LV- and minicircle-derived iPSCs by days 21 and 42, respectively ( Fig. 1a ). By contrast, bioluminescence of the two iPSC lines persisted in immunodeficient NOD/SCID mice, showing a substantial increase over time consistent with teratoma development. These results suggest that the loss of iPSC bioluminescence observed in syngeneic recipients was due to immunological rejection. A consecutive challenge of iPSC-primed mice with syngeneic iPSCs resulted in the accelerated loss of bioluminescence signals, suggesting that antigen-specific immunological memory had developed ( Fig. 1b ). To rule out the possibility that the immune response against iPSCs was elicited by the expression of GFP.Luc + , end point survival of a LV-iPSC line (B6.129.F1) free of these reporter transgenes was also examined [9] . To facilitate graft explantation, these reporter transgene-free iPSCs were implanted subcutaneously in the dorsa of syngeneic and immunodeficient mice and removed after 30 days in vivo . Mouse iPSC grafts explanted from syngeneic mice did not show histological features consistent with teratomas (that is, three germ-layer structure; Supplementary Fig. 2a ), and were significantly smaller in size compared with grafts extracted from immunodeficient animals ( Supplementary Fig. 2b ). To gain additional insight into the quality of the immune response elicited by the syngeneic reporter transgene-free iPSCs, splenocytes from iPSC-primed or naive syngeneic (B6.129.F10) or allogeneic (BALB/c, C57BL/6, and FVB) mice were re-exposed to B6.129.F1 iPSCs ex vivo for 24 h, and IFN-γ production was measured by ELISPOT. Production of IFN-γ by syngeneic mice was statistically undistinguishable to two allogeneic mouse strains (BALB/c and FVB), but significantly lower than the C57BL/6 allogeneic mouse strain ( Supplementary Fig. 2c ). To further examine the effect of IFN-γ on the rejection of these cells, a third iPSC line (C57BL/6) was implanted subcutaneously in the dorsa of syngeneic wild-type or in IFN-γ knockout (IFN-γ −/− ) C57BL/6 recipients. The status of the iPSC grafts was evaluated 30 days post implantation and, as expected, rejection of iPSCs was abrogated in IFN-γ −/− recipients ( Supplementary Fig. 2d ). 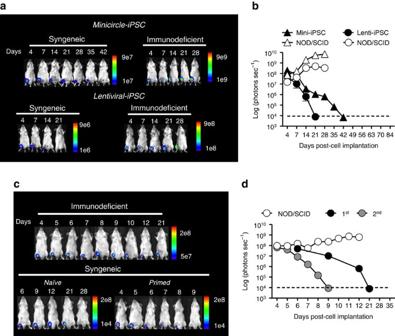Figure 1: Undifferentiated iPSCs derived by LV or genome-integration-free strategies are rejected in syngeneic recipients. LV or minicircle-derived iPSCs expressing GFP and luciferase were injected intramuscularly in syngeneic or immunodeficient recipients, and their survival was monitoredin vivoby bioluminescence imaging (BLI). (a) Representative BLI from one mouse per group demonstrating the longitudinal survival of minicircle- and LV-derived iPSCs in syngeneic and immunodeficient recipients. (b) Mean±s.e.m. bioluminescence of minicircle- versus LV-derived iPSCs in syngeneic and immunodeficient recipients demonstrating a progressive decay in bioluminescence to background levels by 42 days following implantation. After complete decay of bioluminescence signal, mice received a second injection of iPSCs. (c,d) Bioluminescence of iPSCs implanted in primed animals (2nd) had an accelerated decay compared with those receiving the first cell injection (1st). Data are representative of at least 10 animals and 3 independent experiments. Figure 1: Undifferentiated iPSCs derived by LV or genome-integration-free strategies are rejected in syngeneic recipients. LV or minicircle-derived iPSCs expressing GFP and luciferase were injected intramuscularly in syngeneic or immunodeficient recipients, and their survival was monitored in vivo by bioluminescence imaging (BLI). ( a ) Representative BLI from one mouse per group demonstrating the longitudinal survival of minicircle- and LV-derived iPSCs in syngeneic and immunodeficient recipients. ( b ) Mean±s.e.m. bioluminescence of minicircle- versus LV-derived iPSCs in syngeneic and immunodeficient recipients demonstrating a progressive decay in bioluminescence to background levels by 42 days following implantation. After complete decay of bioluminescence signal, mice received a second injection of iPSCs. ( c , d ) Bioluminescence of iPSCs implanted in primed animals (2nd) had an accelerated decay compared with those receiving the first cell injection (1st). Data are representative of at least 10 animals and 3 independent experiments. Full size image The contextual cellularity of iPSC grafts extracted from syngeneic and immunodeficient mice were drastically different ( Supplementary Fig. 3a ). Grafts from syngeneic mice comprised predominantly of pauricellular Matrigel and adipocytes but also contained small areas of undifferentiated iPSCs that could still be detected for up to 14 days post implantation ( Supplementary Fig. 3b ). Surprisingly, large nodules of undifferentiated iPSCs could still be found in teratomas extracted from immunodeficient mice for at least 30 days post-cell implantation ( Supplementary Fig. 3c ). Differences in the contextual cellularity of grafts extracted from syngeneic and immunodeficient mice support the premise that iPSCs, or the early progenitors that spontaneously differentiate upon transplantation, are immunogenic. The ability of iPSCs to elicit immune response in a syngeneic setting was also assessed by measuring ex vivo cytokine responses by splenocytes from mice primed with syngeneic iPSCs. Primed splenocytes cocultured with syngeneic iPSCs released significantly higher abundance of cytokines associated with innate as well as adaptive immune responses compared with naive splenocytes ( Supplementary Fig. 4 ). Although iPSCs did undergo a certain level of differentiation during the 3-day assay, ‘terminal’ differentiation of cells did not occur. Overall, these results support the premise that undifferentiated iPSCs or their early progenitors, which may still carry antigenic determinants from the parental iPSCs, are intrinsically immunogenic and elicit an immune response with strong pro-inflammatory and T-helper 1 elements. Terminal differentiation enables survival of iECs in syngeneic mice GFP.Luc + iPSCs generated by LV-based reprogramming were differentiated in vitro into ECs as previously described [10] , and purified by fluorescence-activated cell sorting (FACS) based on the expression of CD144 and CD31 ( Supplementary Fig. 5a ). Mouse iECs exhibited transcriptome ( Supplementary Fig. 5b ) and surface protein marker ( Supplementary Fig. 5c,d ) profiles that are consistent with ECs. Furthermore, iECs displayed a functional phenotype consistent with ECs, including the production of extracellular matrix material ( Supplementary Fig. 5e ), uptake of low-density lipoprotein (LDL; Supplementary Fig. 5f ) and vasculogenesis ( Supplementary Fig. 5g ). Expression of major histocompatibility complex (MHC) molecules (class-I and class-II) was similar between iECs and AECs ( Supplementary Fig. 5h ). Functionality and tumorigenicity of iECs were also tested in vivo . In a hindlimb ischaemia model, immunodeficient mice were injected with either iECs or vehicle. Engraftment of iECs as well as blood flow in the injured hindlimb were assessed by immunofluorescence staining and laser Doppler perfusion, respectively, 14 days post-cell implantation. iECs successfully engrafted and improved blood perfusion in the hindlimb ischaemia model ( Supplementary Fig. 6a ). Histological evaluation of transplanted murine iECs in the ischaemic hindlimb revealed muscle atrophy and degeneration, but no signs of teratoma formation ( Supplementary Fig. 6b ). Furthermore, immunofluorescence staining for CM-DiI-labelled iPSC-ECs verified the localization and survival of iECs in the ischaemic hindlimbs ( Supplementary Fig. 6c ). Assessment of syngeneic iECs’ immunogenicity was then carried out in vivo and compared with the immunogenicity of the parental iPSC line and to the corresponding syngeneic somatic cell, AEC ( Supplementary Fig. 7 ). To determine the kinetics of cell survival in vivo , cells (1 × 10 6 ) were mixed in Matrigel able to maintain graft integrity in situ , and implanted subcutaneously in the dorsa of syngeneic recipients. Survival was monitored by BLI over 63 days. Unlike iPSCs, bioluminescence signals of iECs and AECs were sustained throughout the entire period ( Fig. 2a,b ). The long-term survival of iECs and AECs in syngeneic recipients provides additional evidence that rejection of iPSCs was not because of alloresponses directed against the reporter transgenes (GFP and luciferase). The survival of iECs and AECs was accompanied by a downregulation of genes previously shown to elicit T-cell-mediated rejection of iPSCs in syngeneic mice [3] , including HORMA domain-containing protein 1 (Hormad1) and zymogen granule protein 16 (Zg16) ( Fig. 2c ). 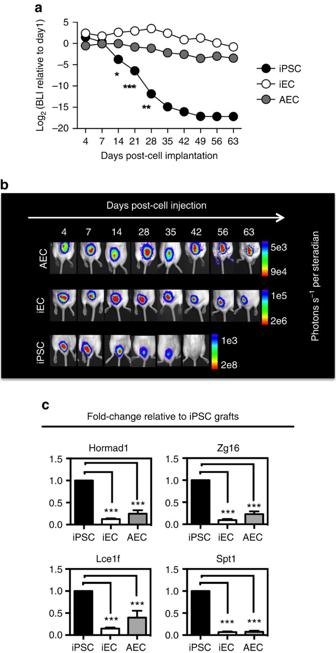Figure 2: Terminal differentiation of iPSCs results in prolonged survivalin vivoand in loss of antigenic determinants. (a) Cellular bioluminescence intensity normalized to day 1 demonstrate a prolonged survival of iECs and AECs relative to iPSCs. (b) Representative bioluminescence images from one animal from each of the three groups over 63 days. Bioluminescence data are representative of two independent experiments with 3–4 animals per group. (c) Gene expression fold-change in iEC and AEC grafts relative to iPSC grafts. Genes previously shown to elicit T-cell-mediated immunological rejection of iPSCs were significantly downregulated in iEC and AEC grafts. Data are representative of mean±s.e.m. of eight biological replicates from three independent experiments. Significance of differences between series of results was assessed using analysis of variance with Tukey for multiple comparisons. *P<0.05, **P<0.01, ***P<0.001. Figure 2: Terminal differentiation of iPSCs results in prolonged survival in vivo and in loss of antigenic determinants. ( a ) Cellular bioluminescence intensity normalized to day 1 demonstrate a prolonged survival of iECs and AECs relative to iPSCs. ( b ) Representative bioluminescence images from one animal from each of the three groups over 63 days. Bioluminescence data are representative of two independent experiments with 3–4 animals per group. ( c ) Gene expression fold-change in iEC and AEC grafts relative to iPSC grafts. Genes previously shown to elicit T-cell-mediated immunological rejection of iPSCs were significantly downregulated in iEC and AEC grafts. Data are representative of mean±s.e.m. of eight biological replicates from three independent experiments. Significance of differences between series of results was assessed using analysis of variance with Tukey for multiple comparisons. * P <0.05, ** P <0.01, *** P <0.001. Full size image Immune response elicited by iECs is similar to the one elicited by self In order to elucidate and compare the nature of the immune response elicited by different cell types, we next implanted subcutaneously lentivirally derived iPSCs devoid of reporter transgenes (B6.129.F1), their progeny iECs and AECs. Cellular grafts were explanted at day 14 and digested enzymatically for cell retrieval. Flow cytometric analysis of the retrieved cells revealed a prominent lymphocytic infiltration in iPSC grafts compared with iEC, AEC and sham (Matrigel only) grafts ( Fig. 3a ). T-cell infiltration was detected in all graft types but was negligible in sham grafts. This suggests that the vehicle used for cell injection had a minimal effect on the immunological response that developed against the different cellular grafts. iECs and AECs elicited similar T-cell infiltration (~4–5% of CD45 + leukocytes), with CD4 + T cells being the most prevalent T-cell type found in these grafts (accounting for ~80% of the CD3 + -infiltrating T cells) ( Fig. 3b,c ). Overall, macrophages (F4/80 + ) represented the majority of the leukocytes infiltrating iECs, AECs and sham grafts ( Supplementary Fig. 8a ). The percentage of FoxP3-expressing CD4 + T cells detected in iPSC grafts was statistically higher than the one found in AECs but indistinguishable from iEC grafts ( Fig. 3d ). At the transcript level, FoxP3 expression in iEC and AEC grafts was elevated compared with iPSC, but these differences did not reach statistical significance ( Supplementary Fig. 8b ). By contrast, a much more hostile immune response was elicited by iPSCs, with significantly higher infiltration of T cells, and CD8 + T cells representing ~50% of the T-cell infiltrates ( Fig. 3b,c ). To further characterize the immunobiology of iECs compared with ‘self’ (AECs) and the parental iPSC lines, mRNA expression of cytokines and cytolytic factors known to be important in rejection responses was measured intragraft. Expression analysis revealed a significant upregulation of granzyme-B, perforin and IFN-γ in iPSC grafts compared with iEC and AEC grafts ( Fig. 3e ). These results suggest that with terminal differentiation, iECs may approach a state of ‘self’ and are tolerated by the immune system. 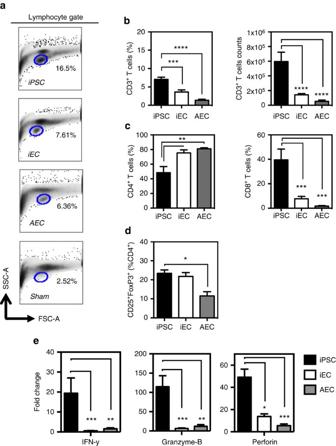Figure 3: Immune response elicited by iECs resembled the one by AECs. Lymphocytic infiltration in cellular grafts was measured by FACS. (a) The iPSC graft displayed marked increase in lymphocytes compared with iEC, AEC and sham grafts. (b) Percentage (left) and absolute counts (right) of infiltrating CD3+T cells was reduced in terminally differentiated iECs and AECs. (c) Helper CD4+T cells were predominant among the T cells infiltrating iEC and AEC grafts. By contrast, cytotoxic (CD8+) T cells were found at a much higher percentage in iPSC grafts. Percentages of CD4+and CD8+cells were calculated from CD3+parental gate. (d) Percentage of FoxP3 expression in CD4+T cells demonstrating higher prevalence in iPSC compared to AEC grafts. (e) Fold-change in gene expression relative to sham grafts demonstrating the differences in immunological milieu intragrafts, with iPSCs having significantly higher mRNA expression of Granzyme-B and Perforin factors compared with iEC and AEC grafts. Data are representative of mean±s.e.m. of eight animals per group from three experiments. Significance of differences between series of results was assessed using analysis of variance with Tukey for multiple comparisons. *P<0.05, **P<0.01, ***P<0.001, ****P<0.0001. Figure 3: Immune response elicited by iECs resembled the one by AECs. Lymphocytic infiltration in cellular grafts was measured by FACS. ( a ) The iPSC graft displayed marked increase in lymphocytes compared with iEC, AEC and sham grafts. ( b ) Percentage (left) and absolute counts (right) of infiltrating CD3 + T cells was reduced in terminally differentiated iECs and AECs. ( c ) Helper CD4 + T cells were predominant among the T cells infiltrating iEC and AEC grafts. By contrast, cytotoxic (CD8 + ) T cells were found at a much higher percentage in iPSC grafts. Percentages of CD4 + and CD8 + cells were calculated from CD3 + parental gate. ( d ) Percentage of FoxP3 expression in CD4 + T cells demonstrating higher prevalence in iPSC compared to AEC grafts. ( e ) Fold-change in gene expression relative to sham grafts demonstrating the differences in immunological milieu intragrafts, with iPSCs having significantly higher mRNA expression of Granzyme-B and Perforin factors compared with iEC and AEC grafts. Data are representative of mean±s.e.m. of eight animals per group from three experiments. Significance of differences between series of results was assessed using analysis of variance with Tukey for multiple comparisons. * P <0.05, ** P <0.01, *** P <0.001, **** P <0.0001. Full size image iPSC immunogenicity is not dictated by reprogramming method In order to determine the potential immunologic effects associated with residual viral DNA in the iPSCs and iEC progeny, an additional integration-free iPSC line was generated. Reprogramming of murine tail fibroblasts was performed using a novel codon optimized mini-intronic plasmid CoMIP expressing the four reprogramming factors such as Oct4, KLF4, Sox2 and c-Myc. MIP-iPSCs were then differentiated to ECs (MIP-iECs) and characterized for endothelial phenotype ( Supplementary Fig. 9 ). Subsequently, MIP-iECs were implanted into syngeneic recipients and grafts were characterized for elements of innate and adaptive immune response such as the percentages of infiltrating immunosuppressive versus pro-inflammatory cell types compared with ECs derived from LV-reprogrammed iPSCs (LV-iECs). Interestingly, our results suggest that transplantation of integration-free non-viral MIP-iECs may not be immunologically advantageous over its LV counterpart. MIP-iECs elicited a 10% higher infiltration of neutrophils compared with LV-iECs ( Fig. 4a ). Among the CD4 + and CD8 + T cells infiltrating MIP-iEC grafts, a higher percentage had an effector memory phenotype (CD44 + ) compared with LV-iEC ( Fig. 4b,c ). Among the CD4 + T cells infiltrating the LV-iEC grafts, a higher percentage of them expressed the activation marker CD69 ( Fig. 4c ), but it is important to note that CD69 expression has also been reported in T regulatory cells (Tregs) known to suppress T-cell proliferation among other suppressive functions [11] . Furthermore, the percentage of CD8 + T cells-expressing granzyme-B, a serine protease released with cytotoxic activity, was significantly higher in MIP-iEC compared with LV-iEC grafts ( Fig. 4d ). Finally, the percentage of FoxP3 + -expressing CD4 + T cells was indistinguishable between MIP- and LV-iEC grafts. Taken together, these data suggest that viral-based methods of iPSC reprogramming may not be any less advantageous than non-viral integration-free-based methods in the context of establishing non-immunogenic iPSC derivatives. We believe that other factors, such as partial reprogramming or genetic instabilities, are likely to have a much more relevant role in dictating the immunological fate of iPSC progeny. 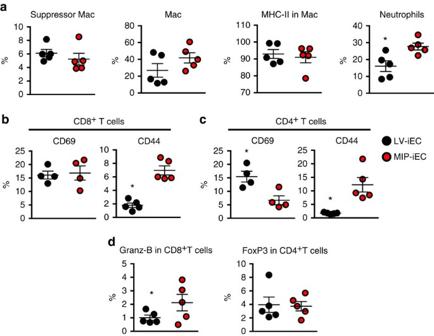Figure 4: FACS analysis of digested LV-iEC and MIP-iEC grafts show differences in immune response elicited in syngeneic recipients. (a) Among the leukocytes infiltrating MIP-iEC and LV-iEC grafts, macrophages (Mac) with either suppressor (CD3−CD11b+CD11c−Gr1+) or activated (CD3−CD11b+CD11c+MHC-II+Gr1−) phenotype were present at similar proportions. MIP-iEC grafts had a significantly higher prevalence of neutrophils (CD3−CD11b−CD11c−Gr1+) compared with LV-iEC. (b,c) A higher percentage of CD8+and CD4+T cells infiltrating MIP-iEC grafts expressed CD44 effector memory marker compared with the ones infiltrating LV-iEC grafts. (d) CD8+T cells infiltrating MIP-iEC grafts had a significantly higher expression of granzyme-B (Granz-B) compared with the ones infiltrating LV-iEC grafts. The percentage of FoxP3+ -expressing CD4+ T cells infiltrating the MIP-iEC and LV-iEC grafts was indistinguishable. Data are representative of mean±s.e.m. of 4–5 animals per group from one experiment. Significance of differences between series of results was assessed using two-tailed unpaired Student’st-test; *P<0.05. Figure 4: FACS analysis of digested LV-iEC and MIP-iEC grafts show differences in immune response elicited in syngeneic recipients. ( a ) Among the leukocytes infiltrating MIP-iEC and LV-iEC grafts, macrophages (Mac) with either suppressor (CD3 − CD11b + CD11c − Gr1 + ) or activated (CD3 − CD11b + CD11c + MHC-II + Gr1 − ) phenotype were present at similar proportions. MIP-iEC grafts had a significantly higher prevalence of neutrophils (CD3 − CD11b − CD11c − Gr1 + ) compared with LV-iEC. ( b , c ) A higher percentage of CD8 + and CD4 + T cells infiltrating MIP-iEC grafts expressed CD44 effector memory marker compared with the ones infiltrating LV-iEC grafts. ( d ) CD8 + T cells infiltrating MIP-iEC grafts had a significantly higher expression of granzyme-B (Granz-B) compared with the ones infiltrating LV-iEC grafts. The percentage of FoxP3+ -expressing CD4+ T cells infiltrating the MIP-iEC and LV-iEC grafts was indistinguishable. Data are representative of mean±s.e.m. of 4–5 animals per group from one experiment. Significance of differences between series of results was assessed using two-tailed unpaired Student’s t -test; * P <0.05. Full size image Terminally differentiated iECs elicit tolerance intragraft In order to better characterize the events that led to the acceptance of iECs, the expression of 84 genes linked to T-cell quiescence and tolerance was quantified in iEC and iPSC grafts. Expression analysis revealed a panel of 19 genes that were significantly upregulated in iEC compared with iPSC grafts ( Supplementary Table 1 ). Hierarchical clustering revealed that some of these genes were part of a prominent aggregate in iEC grafts ( Fig. 5a ). This cluster contained genes known to be negative regulators of T-helper 1 cell-mediated inflammation (STAT3) [12] , [13] , [14] , transducers of apoptosis signals (TNFRSF10b) [15] , mediators of transforming growth factor-β (TGF-β) signalling (Fos) [16] , and potent regulators of adaptive immunity (interleukin-10 (IL-10) and TGF-β) [17] , [18] . More importantly was the striking upregulation of genes that encode the immunoregulatory cytokines IL-10 and TGF-β found in iEC grafts compared with iPSC grafts that was validated on a larger biological sample size ( Fig. 5b ). Furthermore, immunofluorescence staining supported these findings by demonstrating a significant presence of IL-10 in iEC grafts compared with other grafts ( Fig. 5c and Supplementary Fig. 10a ). To rule out the possibility that the abundant IL-10 in iEC grafts originated from cellular infiltrates and not from the iECs themselves, staining of IL-10 was performed in conjunction with an endothelial-specific marker, von Willebrand factor (vWF). No association between IL-10 and vWF was found, suggesting that this cytokine originated from the cellular infiltrates rather than the iECs themselves ( Supplementary Fig. 10b ). Next, to determine the role of IL-10 in promoting iEC acceptance, antibody-based neutralization of IL-10 was performed. Treatment with anti-IL-10 resulted in a reduction of iEC bioluminescence in syngeneic recipients by 3 weeks after cell implantation, suggesting that IL-10 was required for tolerance to iECs ( Supplementary Fig. 11a ). Finally, in order to exclude the possibility that the effects mediated by anti-IL-10 were due to antibody-dependent cell death, anti-IL-10 cytotoxicity to iECs was examined in vitro . Our results showed that anti-IL-10 did not induce iEC cytotoxicity ( Supplementary Fig. 11b ). 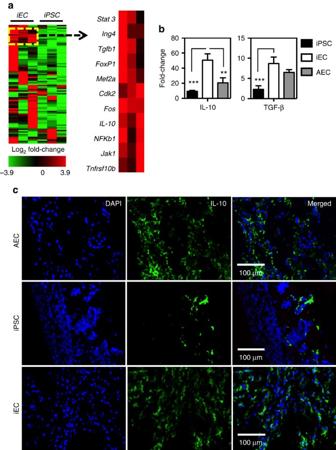Figure 5: iECs elicited activation of a tolerogenic transcriptome network. (a) Hierarchical clustering revealed a group of nine genes (right panel) consistently upregulated in iEC grafts and with similar expression levels. These genes are known members of a pathway involved in regulation of IL-10. Data are representative of three animals per group. (b) Fold-change in gene expression relative to sham grafts confirming the pro-tolerogenic phenotype of iEC and AEC grafts. Data are representative of mean±s.e.m. of 3–4 animals per group from three independent experiments. Significance of differences between series of results was assessed using analysis of variance with Tukey for multiple comparisons. (c) Immunofluorescence staining demonstrating IL-10 abundance in iPSC, iEC and AEC grafts. Quantification of IL-10 expression was performed in five random fields from each graft type ( × 40 magnitude). Data are representative of mean±s.e.m. of a minimum of 1,000 cells from five randomly selected fields. **P<0.01, ***P<0.001. Figure 5: iECs elicited activation of a tolerogenic transcriptome network. ( a ) Hierarchical clustering revealed a group of nine genes (right panel) consistently upregulated in iEC grafts and with similar expression levels. These genes are known members of a pathway involved in regulation of IL-10. Data are representative of three animals per group. ( b ) Fold-change in gene expression relative to sham grafts confirming the pro-tolerogenic phenotype of iEC and AEC grafts. Data are representative of mean±s.e.m. of 3–4 animals per group from three independent experiments. Significance of differences between series of results was assessed using analysis of variance with Tukey for multiple comparisons. ( c ) Immunofluorescence staining demonstrating IL-10 abundance in iPSC, iEC and AEC grafts. Quantification of IL-10 expression was performed in five random fields from each graft type ( × 40 magnitude). Data are representative of mean±s.e.m. of a minimum of 1,000 cells from five randomly selected fields. ** P <0.01, *** P <0.001. Full size image Immune cell infiltrates in differentiated grafts are tolerogenic The tolerogenic effect associated with terminal differentiation of iPSCs on the elicited immune response was further characterized directly on graft-infiltrating immune cells. For this, T cells (CD4 + and CD8 + ) and suppressor macrophages (CD11c − CD11b + Gr1 + ) were isolated from the different grafts by FACS. The expression analysis of a panel of 14 genes, well described in the literature to be associated with suppression of T-cell function and peripheral tolerance [19] , was analysed using the Fluidigm single-cell PCR platform [20] . Expression analysis of the immune cells supported our results by demonstrating that induction of immunological self-tolerance accompanies terminal differentiation of iPSCs ( Fig. 6 ). In the three immune cell types analysed, upregulation of a tolerogenic network of genes was found in T cells and macrophages infiltrating iEC and AEC compared with iPSC grafts. Protein-encoding genes associated with the suppressor function of Tregs and type-1 Tregs (Tr1), such as IL-10 and TGF-β, were consistently upregulated in CD4 + T cell isolated from iEC and AEC grafts. The upregulation of IL-10, which was accompanied by an overexpression of FoxP3 in CD4 + T cells, further strengthens the notion that Tregs may be key factors in modulating acceptance of iECs. Additional protein-encoding genes associated with suppression function as well as anergy of T cells, such as CD39, CD73 (ref. 21 ) and CTLA4 (ref. 22 ), were also similarly upregulated in iECs and AECs. These similarities were particularly evident when comparing AECs to LV-iECs, supporting the flow cytometric results demonstrated in Fig. 5 . Interestingly, MIP-iECs induced a different set of genes to similar levels as the AECs, especially in CD8 + T cells and macrophages. Among these are Egr2 and Egr3 that increase E3 ubiquitin ligases, thereby inhibiting T-cell activation. Furthermore, the induction of PD-1, as well as GRAIL and Itch, which was more evident in MIP-iECs compared with LV-iEC infiltrating CD8 + T cells and macrophages, are known to result in T-cell inhibition [23] , [24] and suppression of pro-inflammatory cytokines [25] . Taken together, our results support the notion that terminal differentiation towards iECs induces a tolerogenic network that is also induced by self. 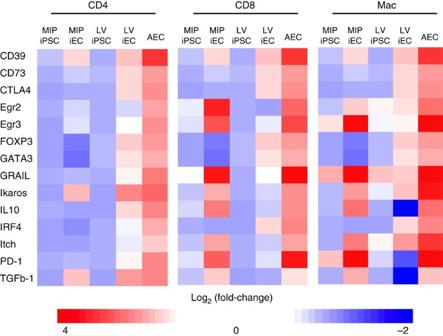Figure 6: Heatmaps illustrating the patterns of expression of genes associated with tolerance and anergy in CD4+T cells, CD8+T cells and suppressor macrophages (Mac; CD3−CD11c−CD11b+Gr1+) extracted from grafts. Fold-change in gene expression of immune cell infiltrates in iEC and AEC grafts relative to undifferentiated iPSC grafts, demonstrating a more tolerogenic and anergic phenotype of immune cells infiltrates from iEC and AEC grafts compared with iPSC grafts. Data are representative of five animals per group. Figure 6: Heatmaps illustrating the patterns of expression of genes associated with tolerance and anergy in CD4 + T cells, CD8 + T cells and suppressor macrophages (Mac; CD3 − CD11c − CD11b + Gr1 + ) extracted from grafts. Fold-change in gene expression of immune cell infiltrates in iEC and AEC grafts relative to undifferentiated iPSC grafts, demonstrating a more tolerogenic and anergic phenotype of immune cells infiltrates from iEC and AEC grafts compared with iPSC grafts. Data are representative of five animals per group. Full size image T-cell clonality of iEC grafts is fundamentally different from iPSCs To further examine similarities among grafts, we next used high-throughput TCR-sequencing analysis of genomic DNA isolated from the tissue grafts to elucidate differences in the clonal structure of T cells infiltrating iPSC, iEC and AEC grafts. We first examined the distribution of CDR3 lengths obtained by sequencing that yielded results very similar to those of a conventional spectratyping method of measuring T-cell repertoire diversity. This produced a restricted skewing in the distribution of CDR3 lengths in iPSC-infiltrating T cells versus iEC- or AEC-infiltrating T cells ( Fig. 7a ). This pattern of restriction in the distribution of CDR3 lengths correlates closely with oligoclonal or monoclonal cells [26] , [27] , [28] . One major limitation of CDR3 spectratyping has been the difficulty in statistically comparing samples or quantifying T-cell clones by sequence identity. We next compared the clonal T-cell repertoire structure in iPSC-, iEC- and AEC-infiltrating T cells. We found that the iPSC-infiltrating T-cell repertoire showed a remarkable expansion of only a few clones when compared with iEC- or AEC-infiltrating T-cell repertoires. We found that the top five dominant T-cell clones accounted for 30–55% of the total TCR diversity of T-cell infiltrates in iPSC grafts, making this T-cell response highly skewed towards a few clones in comparison with the fraction of diversity of the top five clones in iEC (15–20%) or AEC (10–25%) grafts. Therefore, relatively few clones dominated the T-cell infiltrates of iPSC grafts, a pattern that was statistically different from that seen in iEC grafts ( Fig. 7b ; P <0.001; two-tailed unpaired Student’s t -test). Control experiments with splenic samples from the same mice showed no repertoire skewing in the spleens of mice with iPSC grafts, which suggests that the skewed clonality is a property of the grafts themselves and not a biased sampling of the repertoire ( Supplementary Fig. 12 ). These data are consistent with the observation that oligoclonal expansion of a limited number of T-cell clones is a hallmark of adaptive immune recognition that has been characterized as a reproducible feature of tissue rejection, and is regarded as a measure of skewness in TCR repertoire [29] , [30] . 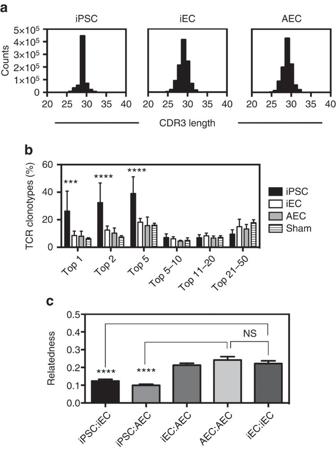Figure 7: T-cell repertoire studies of graft infiltrates. (a) T cells infiltrating iPSC grafts show repertoire restriction. CDR3 length distribution of TCR sequences obtained from a representative syngeneic-rejected iPSC graft (left panel), accepted iEC graft (central panel) and accepted AEC graft (right panel). (b) T cells infiltrating iPSC grafts show a statistically significant expansion of a few dominant T-cell clones compared with iEC- or AEC-infiltrating cells. Results are pooled from two experiments,n=3 mice per group. (c) The T-cell repertoires of iEC and AEC grafts are statistically indistinguishable but different from iPSC repertoires. BCs of relatedness averaged for comparisons within experimental groups. Data are representative of mean±s.e.m. of three animals per group from two independent experiments are reported here. Significance of differences between series of results was assessed using unpaired two-tailed Student’st-test; ***P<0.001, ****P<0.0001. Figure 7: T-cell repertoire studies of graft infiltrates. ( a ) T cells infiltrating iPSC grafts show repertoire restriction. CDR3 length distribution of TCR sequences obtained from a representative syngeneic-rejected iPSC graft (left panel), accepted iEC graft (central panel) and accepted AEC graft (right panel). ( b ) T cells infiltrating iPSC grafts show a statistically significant expansion of a few dominant T-cell clones compared with iEC- or AEC-infiltrating cells. Results are pooled from two experiments, n =3 mice per group. ( c ) The T-cell repertoires of iEC and AEC grafts are statistically indistinguishable but different from iPSC repertoires. BCs of relatedness averaged for comparisons within experimental groups. Data are representative of mean±s.e.m. of three animals per group from two independent experiments are reported here. Significance of differences between series of results was assessed using unpaired two-tailed Student’s t -test; *** P <0.001, **** P <0.0001. Full size image One remaining question is whether the same T-cell clones were expanding within the grafts. We examined this in two ways: the first was to look at how the top 50 T-cell clones within the graft were shared, and the second approach used statistical methods of whole repertoire comparison. We compared all of the mice within each experiment for the number of shared clones in the top 50 by rank order. We found that very few T-cell clones were shared overall ( Supplementary Table 2 ), with iPSC to iPSC comparisons averaging 3.7 shared clones in the top 50 between any two mice within experiments, versus iEC to AEC (11.1 shared clones), iEC to iEC (8.7 shared clones) and AEC to AEC (12.3 shared clones). Importantly, while the exact CDR3 sequence of the top T-cell clones was not the same among grafts for different mice within and between each experiment, the proportion of T-cell expansion was similar. Using an information theory-based metric of similarity, the Bhattacharyya coefficient (BC) of relatedness that takes into account sequence identity and relative frequency of clones between samples [31] , we next examined the similarity in the entire TCR repertoires of T cells infiltrating the different grafts. A comparison of the grafts derived from the same tissue type among mice (iEC versus iEC or AEC versus AEC) showed values between 0.20 and 0.24, whereas the iPSC to iPSC comparison showed a value 0.15–0.18. The comparison of iEC to AEC tissues was statistically indistinguishable from iEC versus iEC, or AEC versus AEC, comparisons ( Fig. 7c ; P =0.66; two-tailed unpaired Student’s t -test). By contrast, comparisons of iPSC to iEC and AEC showed less relatedness with values of 0.12 for iPSC versus iEC and 0.10 for iPSC versus AEC. These results indicate that the TCR repertoire of iPSC-infiltrating T cells is statistically distinguishable from that of iEC- or AEC-infiltrating T cells ( Fig. 7c ). Since AEC and iEC relatedness cannot be distinguished between themselves or from one another, but can be distinguished for comparisons to iPSC, we conclude that the T-cell response to iPSCs is fundamentally different from that of AEC or iEC tissues at a clonal level. Transplantation of tissues derived from autologous iPSCs has the potential to treat many medical conditions, but a major concern for this approach is whether the immune system will accept iPSC-derived terminally differentiated tissues. Recent research has demonstrated that iPSCs retain epigenetic artifacts from the parental cells and from the reprogramming process [32] , [33] . These changes can affect the ability of iPSCs to efficiently differentiate into functional somatic cells, and most importantly, their ability to persist in their differentiated state after terminal differentiation [34] . These factors can have serious implications for the safety and sustainability of iPSC derivatives in vivo , including tumorigenicity [35] and immunogenicity [3] , [36] , [37] . Here we show that iPSCs generated by either LV or genome-integration-free methods are immunogenic in syngeneic recipients, which supports previous findings by Zhao et al. [3] Moreover, our results support recent studies demonstrating that terminal differentiation of iPSCs can result in a loss of immunogenicity [36] , [37] , and show for the first time that terminally differentiated iPSCs elicit immune responses consistent with self-tolerance. Although the lack of rejection of transplanted tissues derived from iPSCs demonstrated here supports findings by Araki et al. [36] and Guha et al. [37] , there are critical differences in the experimental methodologies in these studies with respect to this current study. Here we used a mouse model of autologous transplantation to assess the immunogenicity of cells implanted subcutaneously, similar to the mouse model used by Zhao et al. [3] and Araki et al. [36] We observed that undifferentiated LV iPSCs and genome-integration-free iPSCs elicited a robust immune response in syngeneic recipients that resulted in bioluminescence signal decay over time and failure to form teratomas. However, the identity of the antigenic determinants in iPSC grafts was not addressed in our study, and it remains unclear whether the robust immune response observed was elicited by the iPSCs themselves or by early progenitors that originate from spontaneous differentiation of iPSCs upon transplantation. Our results support the findings described by Zhao et al. [3] , but not by Araki et al. [36] with respect to the rejection of autologous undifferentiated iPSCs. In the study by Guha et al. [37] , cells were implanted in the sub-renal capsule, and rejection of undifferentiated iPSCs was not reproduced. The vascularity and niche of the graft are important factors determining cell survival, immune cell homing and engraftment. The sub-renal capsule is a highly vascularized site that has been vastly used for testing cellular tumorigenicity and has been known to support the growth of tumours that are unable to grow when implanted subcutaneously [38] . Second, the end point for the experiments in the study by Guha et al. [37] was 30 days post-cell implantation. Although histological evidence of cell survival was provided at the study end point, no information that addresses a possible immunogenicity-associated decay in graft viability over the time course of the study is shown. In regards to the immunogenicity of terminally differentiated iPSC progeny, our findings support both Guha et al. [37] and Araki et al. [36] who demonstrate that terminally differentiated cells are immunologically accepted when transplanted syngeneically. Similar to our study, Guha et al. [37] transplanted iPSC derivatives (endothelial, neuronal and hepatocytes) differentiated in vitro , whereas Araki et al. [36] transplanted dermal and bone marrow tissues from highly chimeric mice developed from iPSC and ESC, a strategy that is arguably unrepresentative of a clinical setting. In both studies, grafts were deemed immunogenic based on one end point assessment of cell survival in histological tissue sections collected at 4–5 weeks post transplantation and based on the amount of T-cell infiltration found in grafts. Both studies demonstrated survival of iPSC derivatives at 4–5 weeks post-cell transplantation, with minimal to no T-cell infiltration. However, while the abundance of T-cell infiltration provides important information regarding the involvement of adaptive immune responses on the status of the grafts, relying exclusively on this one parameter to assess the immunogenicity of grafts can be misleading. For instance, regulatory [39] , anergic [40] or exhausted [41] T cells are often found in thriving tumours. These T cells are known to facilitate tumour survival and tumour growth by supporting an immunosuppressive environment. Hence using T-cell infiltration as main evidence for graft immunogenicity may not be ideal [42] , [43] , [44] . In contrast to the undifferentiated parental iPSCs, the endothelial progeny exhibited long-term survival in syngeneic recipients and produced a shift in immunological response consistent with self-tolerance and tissue acceptance. Contrary to previous reports correlating iPSC-derived tissue acceptance to the presence or absence of T-cell infiltration [3] , our results indicate that T-cell infiltration is common to both somatic and iPSC-derived cell grafts. The infiltration of T cells into early grafts may be in response to immune rejection, or in response to the trauma of graft introduction and intragraft cell death of some tissue that invariably occurs. Importantly, while T cells infiltrating grafts early on was a common theme among iPSC, iEC and AEC grafts, we found that the cytokine milieu was very different among grafts. Undifferentiated iPSC grafts possessed hallmark elements of cytotoxic T-cell responses, whereas iEC and AEC grafts elicited a much more ‘benign’ immune phenotype that was dominated by immunoregulatory cytokines such as IL-10 and TGF-β. The highest IL-10 responses were elicited by iEC grafts, suggesting that while the immune acceptance of iEC grafts is similar to AEC grafts, iECs may still have a certain level of antigen disparity with the recipient. Similar situation occurs for tolerance-inducing approaches in solid organ transplantation where IL-10 is needed for the immune protection of MHC-matched, minor-mismatched or major-mismatched grafts in many animal models. In these systems, the production of IL-10 in the graft environment is critical for peripheral tolerance and graft acceptance. A key question in the field is how similar to “self” must a graft be in order to be tolerated by the immune cells; our work shows that iECs are sufficiently similar to ’self’ tissue to be tolerated. But the exact mechanism(s) that led to the differences in tolerogenic response elicited by iEC and AEC grafts will require further investigation. It is important to also consider that the self-tolerogenic response elicited by terminally differentiated ECs may also facilitate the survival of cells with oncogenic potential. Thus, the realization that self-tolerance may potentiate tumorigenesis of autologous iPSC-derived cells needs to be carefully considered and evaluated before clinical translation. Finally, the percentage of FoxP3-expressing CD4 + T cells detected in iPSC grafts was statistically higher than the one found in AECs but was indistinguishable from iEC. Increases in FoxP3 expression have been noted in active immune rejection and may not be as reliable as a marker of tolerance in this setting as measuring effector molecules [45] , [46] . Similarities in FoxP3 expression between iEC and AEC grafts were present at the mRNA level in total graft tissue as well as in T-cell infiltrates. We also examined the TCR clonal structure of rejecting tissue. Until very recently, oligoclonal and monoclonal T-cell responses in tissue rejection were measured using spectratyping and V- and J-chain usage restriction, which is a relatively low-resolution method for tracking specific T-cell clones mediating rejection. Alternatively, exhaustive studies have identified specific antigen responses in allogeneic transplants. In some of these cases, the expansion of dominant allo-reactive T cells was found. Using a higher-resolution method for tracking clonal T-cell responses of repertoire sequencing, we found that relatively few oligoclonal T cells are greatly expanded in iPSC graft infiltrates versus AEC or iEC grafts. This suggests that iPSC graft-infiltrating repertoire has a pattern of immune rejection. Importantly, the same T-cell clones do not appear to dominate tissue rejection responses, likely because iPSCs can rapidly and stochastically divide into any number of differentiating tissues and the resulting T-cell responses are variable. Our analysis offers novel ways to use TCR repertoire sequencing to help distinguish graft rejection from graft tolerance. Although there is potential for PCR bias in the TCR amplification, all experiments were performed such that all samples from each group—iPSC, iEC, AEC and sham control—were processed at the same time and had the same primers and reagents. Given that the iPSC grafts clearly had different dominant clonal sequences among themselves in the grafts, we believe that these results are less likely because of the artificial overstating of a clone that appears in iPSC grafts and not in other grafts. In addition, control experiments with splenic samples from the same mice showed no repertoire skewing in the spleens of mice with iPSC grafts, which suggests that the skewed clonality is a property of the grafts themselves and not a biased sampling of the repertoire. Although correction of PCR amplification bias should be a goal of the field, so far this is an underappreciated point in the current literature. Researchers are still trying to optimize methods to control for PCR amplification bias and disseminate these methods that is a highly innovative approach not previously available and not tested for murine or other animal models, as recently pointed out by the study by Carlson et al. [47] PCR amplification bias is very important for questions such as the detection of minimal residual disease, and statistical analysis can now be applied without bias correction as discussed in Meyer et al. [48] Overall, our statistical analysis explicitly examines the probability of a chance event that a specific clone is somehow amplified better in one sample versus another, but our P values suggest that this is not the case. In summary, our results indicate that iPSC-derived tissues can be accepted by the immune system without immunosuppressive therapy in a tolerant manner very similar to autologous tissues. Our results also suggest that viral-based reprogramming of iPSCs may not be critical in dictating downstream immunogenicity of iPSC progeny. Before clinical translation of iPSC-derived cellular therapy, it will be critical to determine the level of permissible dissimilarity that allows these therapeutic cells to be seen as ‘self’ in autologous transplantation settings. Moreover, establishing the ‘ground’ state of iPSCs (at the epigenome, genome, and proteome levels) required for derivation of safe cellular therapeutics that act as ‘self’ upon transplantation is imperative for the eventual clinical adoption of this technology. Mice Six- to eight-week-old female FVB, NOD-SCID IL2Rgamma null , C57BL/6 and IFN −/− were obtained from The Jackson Laboratory. B6.129.F1 females were obtained from Taconic. Transgenic FVB mice expressing luciferase and GFP were generated at the transgenic animal facility in the Department of Pathology at Stanford University by pronuclear injection of the reporter gene construct. Mice were maintained at the Stanford University Research Animal Facility in accordance with Stanford University’s Institutional Animal Care and Use Committee guidelines. Derivation and characterization of iECs iECs were derived using a three-dimensional approach with modifications [10] . In brief, to initiate differentiation, iPSCs were cultured in ultra-low, non-adhesive dishes to form embryoid body (EB) aggregates in EBM2 media (Lonza) in the absence of leukaemia inhibitor factor. After 4 days of suspension culture, the EBs were reattached onto 0.2% gelatin-coated dishes and cultured in EBM2 medium supplemented with vascular endothelial growth factor (VEGF)-A165 (50 ng ml −1 ; PeproTech). After 3 weeks of differentiation, single-cell suspensions were obtained using a cell dissociation buffer (Life Technologies, Grand Island, NY, USA) and labelled with APC-conjugated CD31 (eBiosciences) and PE-conjugated CD144 (BD Biosciences) anti-mouse antibodies. iECs were purified by FACS of CD31 + CD144 + population. iECs were maintained in EBM2 media supplemented with recombinant murine vascular endothelial growth factor (50 ng ml −1 ). Isolation of AECs B6.129.F10 mice were killed and the ascending and descending aorta segments were harvested. Aorta was cleaned from surrounding adipose tissue under dissecting microscope. Subsequently, aorta was mechanically and enzymatically dissociated in Collagenase II (1 mg ml −1 ) by incubating at 37 °C for 45 min. The digestion mix was triturated every 10 min to ensure complete dissociation. At the end of 45 min, the cell suspension was filtered through a 70-μm strainer to attain a single-cell suspension. Cell suspension was centrifuged at 1,200 r.p.m. for 5 min. The pellet obtained was subjected to red blood cell lysis, followed by a wash with phosphate-buffered saline (PBS) and centrifugation at 1,200 r.p.m. for 5 min. The pellet enriched in ECs was immediately seeded on a 0.2% gelatin-coated plate in EGM2 media (Lonza). After 2 weeks of in vitro expansion, ECs were further purified by FACS based on the expression of CD144 and CD31. Cell graft implantations Cell injection was conducted under the guidelines of Stanford University Administrative Panel of Laboratory Animal Care. Mice were placed in an induction chamber and anaesthesia was induced with 2% isoflurane (Isothesia, Butler Schein) in 100% oxygen with a delivery rate of 2 l min −1 until loss of righting reflex. Cells (1 × 10 6 ) were mixed in 200 μl BD Matrigel High Concentration (1:2; BD Biosciences) and injected subcutaneously in the lower dorsa of mice using a 28-G syringe. In vivo BLI Transplanted cell survival was longitudinally monitored via BLI using the Xenogen In Vivo Imaging System (Caliper Life Sciences). In brief, D -luciferin (Promega) was administered intraperitoneally at a dose of 375 mg kg −1 of body weight. Animals were placed in a light-tight chamber, and photons emitted from luciferase-expressing cells were collected with integration times of 5 s to 2 min, depending on the intensity of the bioluminescence emission. BLI signal was quantified in maximum photons s −1 cm −2 per steradian and presented as Log 10 (photons s −1 ). Graft explantation and cell isolation Grafts were explanted, chopped into small fragments and digested with Liberase (27 WU ml −1 ; Roche, Indianapolis, IN, USA) and DNase I (0.1%; Roche) in Dulbecco’s modified Eagle medium (DMEM) media at room temperature for 30 min followed by incubation at 37 °C for 15 min. Digested grafts were passed through a 100-μm strainer and centrifuged at 300 g for 10 min at 4 °C. Cells were counted and prepared for flow cytometry or snap frozen for RNA and DNA extractions. Flow cytometric analysis of graft-infiltrating lymphocytes Fluorophore-conjugated monoclonal antibodies against mouse CD3, CD4, CD8, CD25, FoxP3, CD11c and NK1.1 (1:100; BD Bioscience or eBioscience) were used in various combinations to stain cells extracted from grafts. For staining, 1 × 10 6 cells were used. The Fc receptor was blocked by CD16/32 antibody. Cells were fixed and permeabilized using BD Cytofix/Cytoperm fixation and intracellular staining was performed. Cells were assayed using a LSRII flow cytometer (BD Biosciences) and further analysed with FlowJo software (Tree Star, Ashland, OR, USA). T-cell tolerance and anergy PCR array Cell grafts harvested from syngeneic recipients 14 days post implantation were enzymatically dissociated to a single-cell suspension and washed with PBS for total RNA extraction by Qiagen RNeasy Mini kit. The RT2Profiler PCR Array kits were purchased from SA Bioscience Corporation (Frederick, MD, USA), and all assay procedures were conducted in accordance with the user kit manual. In brief, 1 μg of total RNA from iPSCs or iECs was transcribed into first strand cDNA and loaded into 96-well PCR array plates with 25 μl quantitative PCR master mix per well. After performing quantitative PCR, resulting threshold cycle values for all genes were exported into the company-provided data analysis template Excel files for comparison of gene expression between iPSC and iEC grafts. Immunocytochemistry for iEC characterization Primary antibodies for mouse vWF (1:150; Millipore), laminin (1:100; Abcam, Cambridge, MA, USA) and CD144 (1:100; Abcam) were used for iEC characterization. iECs were grown in 0.2% gelatin-coated coverslips and fixed in 4% paraformaldehyde when they reached 80% confluence. Before immunostaining, cells were blocked with 1% BSA for 1 h at room temperature. Subsequently, primary antibodies were maintained overnight at 4 °C. Coverslips were washed in PBS and incubated with goat anti-rabbit Alexa Fluor 594 (Invitrogen) for 1.5 h at room temperature. For intracellular staining of vWF, cells were permeabilized with 0.2% Triton X-100 then subjected to BSA blocking and incubation with the antibody diluted in 1% BSA and 0.1% Triton X-100. Confocal images were taken using Carl Zeiss, LSM 510 Meta (Göttingen, Germany) using a × 63 plan apochromat (oil) objective microscope. Images were analysed using the ZEN software (Carl Zeiss). LDL uptake Acetylated LDL (ac-LDL) uptake was performed by incubating iEC monolayers in rhodamine-conjugated ac-LDL (10 μg ml −1 ; Biomedical) for 4 h at 37 °C. Subsequently, the medium was removed and cells were washed with a probe-free medium and harvested for flow cytometric characterization. Histological analysis Grafts were harvested and cryo-embedded directly in Tissue Tek O.C.T. (Sakura Finetek) or fixed in 10% buffered formalin overnight after which they were transferred to a 15% w/v sucrose solution until tissue processing and paraffin embedding. Multiple 5 μm tissue sections from each sample were cut at mid-teratoma and stained with haematoxylin and eosin for histological analysis. Frozen blocks were mounted on a Leica cryostat CM3050 S (Leica Microsystems) and 8 μm sections were transferred to Superfrost/Plus adhesive slides (Fisher brand) and stored at −80 °C. For characterization of cellular contexture of grafts, a pathologist, blinded to the to sample assignment, measured the total surface area of each graft cross-section, assigned lineage differentiation to each of the morphologic components, and determined the representation of each component as a percentage of the total mid-tumour cross-sections area. IL-10 immunoassaying Immunostaining was performed using antibodies against IL-10 (1:100; Abcam) and Alexa-488-conjugated (Life Technologies) secondary antibodies (1:1,000). Frozen sections were fixed in acetone followed by blocking in 5% horse serum for 60 min at room temperature. Sections were then incubated with primary antibody in blocking solution overnight at 4 °C. Nuclei were stained with Hoechst 33342 (Life Technologies). Fluorescent images were taken with a Leica SP2 AOBS (Acousto-Optical Beam Splitters) Confocal Laser Scanning Microscope with × 20, × 40 and × 63 oil objectives. For resolution of nuclei-dense regions, Z-stacked confocal images were rendered into three dimensions using Volocity 6.0.1 software. For IL-10 + cell counts, one independent blinded observer examined five random fields at × 40 magnitude. Quantification of IL-10 staining was determined by planar association of stain and nuclei. IL-10 neutralization in vivo Neutralization of IL-10 was performed using anti-IL-10 antibody (JES5-2A5, BioXCell) or isotype control anti-Rat IgG1 (BioXCell). Mice received 250 μg of antibody intraperitoneally on days −1, 1, 3, 6, 9 and 12 relative to cell implantation. Cell viability assay Cell viability upon treatment with JES5-2A5 antibody was analysed using an XTT-based in vitro toxicology assay kit (Sigma-Aldrich). Cells were grown in a 96-well plate (Corning) to about 50% confluency, and subsequently subjected to 48 h treatment of different concentrations of JES5-2A5 antibody. During the last 12 h, control cells were treated with 50 nM Antimycin A, a Complex III inhibitor of the mitochondrial electron transport chain, as a positive control for cytotoxicity. Cells at a final density of ~80% were incubated for 4 h in the presence of a 20% XTT reagent diluted in culture medium, protected from light. Absorbance at 450 nm was measured using a plate-reader (Promega). Derivation and culture of non-viral murine iPSCs Murine tail tip fibroblasts of mice were dissociated and isolated with collagenase type IV (Life Technologies) and maintained with DMEM containing 10% fetal bovine serum, L-glutamine, 4.5 g l −1 glucose, 100 U ml −1 penicillin and 100 μg ml −1 streptomycin at 37 °C, 20% O 2 and 5% CO 2 in a humidified incubator. Murine fibroblasts (1 × 10 6 m) were then reprogrammed using a CoMIP (10–12 μg of DNA) expressing the four reprogramming factors Oct4, KLF4, Sox2 and c-Myc using the Neon Transfection system (unpublished data). After transfection, fibroblast were plated on a MEF feeder layer and kept in fibroblast media with the addition of sodium butyrate (0.2 mM) and 50 μg ml −1 ascorbic acid. When ESC-like colonies appeared, media was changed to murine iPSC media containing DMEM, 20% fetal bovine serum, L-glutamine, non-essential amino acids, β-mercaptoethanol and 10 ng ml −1 leukemia inhibitory factor. After two passages, the murine iPSCs were transferred to 0.2% gelatin-coated plates and further expanded. With every passage, the iPSCs were sorted for the murine pluripotency marker SSEA-1 using magnetic-activated cell sorting. Immunofluorescence staining of cultured cells Cells were fixed with 4% paraformaldehyde for 20 min, permeabilized with 0.2% Triton X-100 in PBS for 30 min and blocked with serum in PBS for 1 h. Cells were then stained with appropriate primary antibodies and Alexa Fluor-conjugated secondary antibodies (Life Technologies) and costained with 4′,6-diamidino-2-phenylindole (DAPI) (Vector Laboratories, Burlingame, CA, USA). The primary antibodies for CD31 and CD144 (Abcam) were used in the staining. All murine iECs were also incubated with 10 μg ml −1 DiI ac-LDL (Life Technologies) at 37 °C for 6 h. After washing twice with PBS, DiI ac-LDL uptake was detected with fluorescence microscopy. Imaging was performed on a Leica DFC500 inverted microscope. Quantitative real-time PCR analysis Total RNA was purified from iPSCs and teratomas using RNeasy Mini kit (Qiagen, CA, USA). RNA (1 μg) was reverse transcribed using a high-capacity cDNA transcription kit (Applied Biosystems), followed by high-throughput quantitative gene expression analysis using the Syber green-based assay system on the StepOne Plus Realtime PCR platform (Applied Biosystems). Primer sequences for Hormad1, Zg16, Lce1f and Spt1 were the same as previously described [3] . GAPDH was used as the internal control gene for all samples and the ΔΔ C t method was used to calculate fold-change of gene expression. For characterization of the intragraft immunological milieu, Taqman-based real-time PCR was carried out using the same platform as described above. The following Taqman probes were used: IFN -γ (Mm01168134_m1), FoxP3 (Mm00475162_m1), GAPDH (Mm99999915_g1), IL-10 (Mm00439614_m1), TGF-β1 (Mm01178820_m1), Perforin (Mm00812512_m1) and granzyme-B (Mm00442834_m1). For characterization of iECs, the following Taqman probes were used: vWF (Mm00550376_m1), CD144 (Mm03053719_s1), and FLK1 (Mm01222421_m1). TCR sequencing Genomic DNA was obtained from explanted grafts using Qiagen DNA extraction kits (Qiagen). Multiplex sets of sequencing tagged primers were used to PCR-amplify all the members of the TCRβ repertoire present in a sample using multiplexed primers consisting of 21 V segment primers and 11 J segment primers designed by Gigagen Inc. (South San Francisco, CA, USA). Pooled (AEC, iPS, iEC and sham) samples were run on an Illumina MiSeq (Illumina, San Diego, CA, USA) to a depth of 2 million sequence reads. The sample sorted fastq files were analysed using the custom coded in Practical Extraction and Report Language (PERL) with bash scripting automation. Only error-free TCR sequences occurring at >2 copies were included in analysis. The BC measures the amount of overlap between two statistical samples, each with a finite number of distinct partitions and probabilities, corresponding to unique clonotypes and their frequencies. It is calculated as: where f j, 1 and f j, 2 are the frequencies of clonotype j in samples 1 and 2, respectively, and n is the number of unique clonotypes present across samples 1 and 2. A BC of 1 between two Rep-Seq samples would mean that the samples are identical in number, sequence and frequency of unique clonotypes. A value of 0 would mean that no clonotypes are present in both samples, although a value of 0.0 would not be informative about the number of clonotypes or frequencies in either sample. The coefficient was calculated using customize PERL scripts. Statistical evaluation of the comparison of Bhattacharya distances was performed using a standard T -test with GraphPad Prism. Statistical methods Differences between groups were assessed by two-way analysis of variance or Student’s t- test using GraphPad Prism software. Bar graphs represent the mean and s.e.m. for each group. Accession codes: Sequencing data has been deposited in NCBI Biosample under accession number SAMN02708924. How to cite this article: de Almeida, P. E. et al. Transplanted terminally differentiated induced pluripotent stem cells are accepted by immune mechanisms similar to self-tolerance. Nat. Commun. 5:3903 doi: 10.1038/ncomms4903 (2014).